The NIN transcription factor coordinates CEP and CLE signaling peptides that regulate nodulation antagonistically Legumes tightly regulate nodule number to balance the cost of supporting symbiotic rhizobia with the benefits of nitrogen fixation. C-terminally Encoded Peptides (CEPs) and CLAVATA3-like (CLE) peptides positively and negatively regulate nodulation, respectively, through independent systemic pathways, but how these regulations are coordinated remains unknown. Here, we show that rhizobia, Nod Factors, and cytokinins induce a symbiosis-specific CEP gene, MtCEP7 , which positively regulates rhizobial infection. Via grafting and split root studies, we reveal that MtCEP7 increases nodule number systemically through the MtCRA2 receptor. MtCEP7 and MtCLE13 expression in rhizobia-inoculated roots rely on the MtCRE1 cytokinin receptor and on the MtNIN transcription factor. MtNIN binds and transactivates Mt CEP7 and MtCLE13 , and a NIN Binding Site (NBS) identified within the proximal MtCEP7 promoter is required for its symbiotic activation. Overall, these results demonstrate that a cytokinin-MtCRE1-MtNIN regulatory module coordinates the expression of two antagonistic, symbiosis-related, peptide hormones from different families to fine-tune nodule number. About 60 million years ago, members of the Fabaceae (legume) plant family evolved the ability to enter into a symbiotic relationship with nitrogen-fixing soil bacteria, generically called rhizobia, to build a dedicated organ on their root system, the root nodule [1] . When mineral nitrogen is limiting in soils, symbiotic rhizobia can provide the nitrogen necessary to support plant growth from the unlimited atmospheric reservoir, thus giving legume plants a competitive advantage in these environments. Legume root nodules initiate following the secretion of rhizobial Nod factor (NF) signals that are perceived at the root epidermis, preferentially in a susceptible region located above the root apical meristem in compatible host plants [2] , [3] , [4] . This symbiotic partner recognition triggers a signaling cascade that activates the rhizobial infection of root hairs and subsequently the formation of infection threads (ITs) that grow toward root inner cortical cells. Simultaneously, rhizobium and NF perception (NFP) at the root epidermis activate cell divisions mostly in the inner cortical and pericycle cells to initiate a nodule organ primordium [5] , [6] , which is reached by growing ITs filled with rhizobia. This primordium then differentiates into a root nodule to accommodate the nitrogen-fixing rhizobia. The legume plant then provides carbon sources to rhizobia, as well as a low oxygen environment that is required to enable the bacterial nitrogenase to fix atmospheric nitrogen in root nodules. Rhizobial NF signaling in host plant roots rapidly activates the transcription of early nodulation genes such as ENOD11 (for early nodulin 11 ) in the root epidermis. ENOD11 expression then follows IT progression from the root epidermis to the cortex [7] . Therefore, ENOD11 can be considered as a marker for early symbiotic signaling activation and rhizobial infections [8] . Downstream of NF signaling activation, nodule organogenesis requires cytokinin since cytokinin receptor loss-of-function mutants (e.g., lotus histidine kinase 1 [ lhk1 in Lotus japonicus ] or cytokinin response 1 [ cre1 in Medicago truncatula ]) have a reduced nodulation capacity [9] , [10] , [11] , [12] , [13] . Consistently, the constitutive activation of LHK1 in the L. japonicus spontaneous nodule formation2 ( snf2 ) mutant triggers ectopic cortical cell divisions and spontaneous nodulation in the absence of rhizobia [14] . Cytokinin additionally negatively regulates rhizobial infections or NF signaling in L. japonicus and M. truncatula , respectively [10] , [15] , [16] , [17] . Combined molecular and genetic analyses allowed the identification of genes critical for nodule initiation. Among those, a L. japonicus mutant defective in rhizobial entry into root hairs was affected in the nodule inception (NIN) transcription factor (TF) [18] . NIN expression is rapidly activated after the perception of NF, and a root hair-specific transcriptomic analysis suggests that NIN regulates rhizobial infections [18] , [19] , [20] . Accordingly, NIN is required for the initiation of symbiotic infections in root hairs [21] . In addition, NIN expression is induced rapidly by cytokinin depending on the CRE1 receptor [9] , [11] , and the constitutive expression of NIN in L. japonicus is sufficient to activate ectopic cortical cell divisions in the absence of rhizobia [22] . Furthermore, M. truncatula NIN also restricts the extent of ENOD11 expression in the root rhizobial susceptible zone, and nin presumptive null mutants are impaired in IT formation [18] , [23] . The L. japonicus nin daphne allele, however, shows a non-nodulation phenotype associated with a high number of ITs, indicating that the root zone susceptible for rhizobial infection is enlarged in daphne [24] . The daphne nodulation phenotype is associated with a broader epidermal expression of NIN than in the wild type (WT). In M. truncatula , a daphne-like mutant was recently identified, and the NIN coding sequence expressed from a 5 kb proximal NIN promoter region was sufficient to rescue its hyperinfection phenotype, even though this region was not sufficient to restore nodule organogenesis [25] . Indeed, an additional remote cis -regulatory sequence located 18 kb upstream from the NIN gene start codon was required to complement nodule organogenesis of the daphne-like nin mutant. Hence, NIN coordinates NF responses, rhizobial infection, and nodule organogenesis. NIN additionally controls nodule number, since this TF triggers the expression of secreted Clavata3/embryo surrounding region (CLE) signaling peptides involved in the negative autoregulation of nodulation (AON) pathway [26] . These AON signaling peptides are referred to as CLE12 and CLE13 in M. truncatula , CLE-RS (CLE-root signal) 1, CLE-RS2, and CLE-RS3 in L. japonicus , and RIC (rhizobium-induced CLE) in Glycine max [27] , [28] , [29] , [30] , [31] . CLE-RS1 and CLE-RS2 genes are expressed within 1 day post rhizobial inoculation [32] , and both in L. japonicus and G. max , NIN directly binds promoters and activates the expression of these nodulation-related CLE peptide-encoding genes to initiate the long distance (systemic) AON pathway [31] , [32] . Shoot-to-root AON signals then generate a negative feedback loop on NIN expression, thus allowing a homeostatic regulation of the root nodule number [32] . CLE peptides produced in roots inoculated with rhizobia are proposed to be translocated through the xylem vasculature to the shoot where they are perceived by the leucine-rich repeat-receptor like kinase (LRR-RLK) SUNN (super numeric nodules) in M. truncatula or HAR1 (hypernodulation and aberrant root 1) in L. japonicus [33] , [34] , [35] , [36] . The activation of this systemic root-to-shoot pathway leads to the production of shoot-to-root signals that further inhibit the formation of new nodules in roots [2] , [16] , [37] . Beside this negative systemic AON pathway, C-terminally encoded peptides (CEPs) regulate an independent systemic pathway in M. truncatula that promotes rhizobial infections and nodule number [3] , [38] , [39] , [40] , [41] . Low nitrogen and nitrogen starvation enhances the expression of several Arabidopsis thaliana and M. truncatula CEP genes, indicating that activation of the CEP pathway is tightly linked to nitrogen deficiency [37] , [38] , [42] . CEP peptide activation of nodulation depends on the LRR-RLK compact root architecture 2 (CRA2) acting in shoots [39] . Indeed, the exogenous application or overexpression of M. truncatula CEP1 peptides promote nodulation [3] , [38] , [40] , and cra2 mutants form a reduced number of nodules [39] , [41] . The closest homolog of CRA2 in Arabidopsis, CEPR1 (CEP receptor 1), directly binds CEP peptides and mediates an N-demand systemic signaling pathway [43] and the allocation of nutrients to roots [44] . In M. truncatula , a functional redundancy between CEP peptide-encoding genes required for the regulation of nodulation is anticipated since an RNA interference (RNAi) silencing of CEP1 and CEP2 genes did not reveal any nodulation phenotype, despite an increased lateral root phenotype was clearly observed, validating the efficient knockdown of these genes [38] . Symbiosis-specific CEP genes required for the positive control of root nodulation thus remain to be characterized. In this study, we identify a M. truncatula CEP peptide-encoding gene, MtCEP7 , with a unique symbiotic expression pattern. MtCEP7 is induced rapidly in response to rhizobia or by short-term treatments with NF or cytokinin. MtCEP7 expression depends on the MtCRE1 cytokinin receptor and on the MtNIN TF, and we show that MtNIN binds to the MtCEP7 and MtCLE13 promoters and can transactivate their expression. The addition of MtCEP7 peptides promotes nodulation systemically through the MtCRA2 receptor, and consistently, MtCEP7 downregulation reduces nodule number and the number of rhizobial infections. MtCEP7 expression is rapidly induced by rhizobia in the root epidermis and the 5 kb MtNIN promoter is sufficient to restore MtCEP7 and MtCLE13 induction by rhizobia, indicating that MtNIN activity induces the coordinated expression of specific nodulation-related signaling peptides from two different families. Strikingly, the expression of the MtCEP7 gene driven by MtCLE13 promoter sequences mitigates the onset of AON, suggesting that the balance between MtCLE13 and MtCEP7 expression might determine the number of successful infections in M. truncatula roots. Overall, these results indicate that a single cytokinin/MtCRE1/MtNIN regulatory module regulate two antagonistic, nodulation-related, signaling peptides, which allows a dynamic fine-tuning of the level of rhizobial infection and of the number of nodules. MtCEP7 is induced by rhizobium, NFs, and cytokinin To identify CEP peptides involved in the regulation of symbiotic nodulation, we analyzed CEP gene expression in response to rhizobia as well as to NF or cytokinin signals that are required for nodule initiation. Only MtCEP7 expression was induced within 1 day post inoculation (dpi) and in response to a short-term treatment with NFs (10 −9 M, 3 h), whereas the other CEP genes were either weakly regulated or showed a reduced expression (e.g., MtCEP5 and MtCEP8 ; Fig. 1a, b ). An independent validation of the NF-dependent regulation of MtCEP7 expression was obtained by using a mutant affecting the previously characterized NFP gene [45] . Indeed, the fast rhizobial induction of MtCEP7 expression was abolished in the nfp mutant, as expected (Supplementary Fig. 1 ). Fig. 1: Expression of CEP peptide-encoding genes in response to rhizobia, Nod factors, or cytokinins. a Expression analysis of CEP genes in wild-type (WT) roots 1 day post rhizobial inoculation (1 dpi). qRT-PCR was used to measure the CEP gene expression levels, normalized relative to uninoculated roots. To highlight fold changes, the dotted line corresponds to a ratio of 1. Data points from four biological replicates are plotted as open circles ( n = 8). b Expression analysis of CEP genes in WT roots in response to a Nod factor (NF) 10 −9 M treatment for 3 h. qRT-PCR was used to measure the CEP expression levels in treated roots. The results were normalized relative to untreated roots. To highlight fold changes, the dotted line corresponds to a ratio of 1. Data points from six biological replicates are plotted as open circles ( n ≥ 11). c Expression analysis of CEP genes in WT roots in response to a cytokinin (BAP 10 −7 M) treatment for 3 h. qRT-PCR was used to measure the CEP gene expression levels in treated roots. The results were normalized relative to untreated roots. To highlight fold changes, the dotted line corresponds to a ratio of 1. Data points from four biological replicates are plotted as open circles ( n ≥ 8). In a – c , center lines show the medians; box limits indicate the 25th and 75th percentiles as determined by the R software; whiskers extend 1.5 times the interquartile range from the 25th and 75th percentiles, outliers are represented by dots; and crosses represent sample means. Mann–Whitney test was used for each gene to assess significant differences between treated and control conditions, as indicated by asterisks (* α < 0.05; ** α < 0.01; *** α < 0.001). Full size image CEP gene expression was then analyzed in response to a 3-h treatment with another signal that promotes nodule initiation, namely, cytokinin (benzyl amino purine [BAP] 10 −7 M). Once more, only MtCEP7 was induced, whereas the expression of most of CEP genes (i.e., MtCEP2 , MtCEP4 , MtCEP5 , MtCEP6 , and MtCEP8 ) was reduced (Fig. 1c ). These analyses therefore highlight that MtCEP7 has a unique expression pattern, being rapidly induced by rhizobia as well as by the two key signals required for nodule initiation, NFs and cytokinin. MtCEP7 symbiotic expression relies on MtCRE1 and MtNIN As the role of cytokinin in early nodulation relies predominantly on the MtCRE1 cytokinin receptor [11] , [12] , we investigated whether the rhizobia-, NF- and cytokinin-regulated MtCEP7 expression depended on MtCRE1. The induction of MtCEP7 by these treatments was strongly reduced in the cre1 mutant (Fig. 2a–c ). These results indicate that the rhizobia, NF, and cytokinin upregulation of MtCEP7 expression depends on the MtCRE1 cytokinin receptor, which further links MtCEP7 to rhizobial infections. As the induction of MtCLE13 in response to cytokinin depended on MtCRE1 [46] , its expression was tested in response to a 24-h treatment with rhizobia and to a 3-h treatment with NFs or cytokinins. As expected, MtCLE13 expression was induced by these treatments and was diminished in the cre1 mutant (Fig. 2a–c ). Fig. 2: Rhizobia, Nod factor, and cytokinin regulation of CEP7 and CLE13 expression relies on the CRE1 cytokinin receptor and on the NIN transcription factor. a – c Expression analysis of the MtCEP7 and MtCLE13 genes in wild-type (WT) or cre1 mutant roots in response to a 1 day post rhizobial inoculation (1 dpi) ( a ), to a Nod factor (NF) 10 −9 M treatment for 3 h ( b ), or to a cytokinin (BAP 10 −7 M) treatment for 3 h ( c ). qRT-PCR was used to measure the gene expression levels in treated roots, normalized relative to untreated roots. Data points from four biological replicates are plotted as open circles ( n ≥ 8). d – f Expression analysis of MtNIN , MtCLE13 , and MtCEP7 genes in WT roots in response to a rhizobial inoculation 1 dpi ( d ), to an NF 10 −9 M treatment for 3 h ( e ), or to a cytokinin (BAP 10 −7 M) treatment for 3 h ( f ). qRT-PCR was used to measure the gene expression levels in treated roots, normalized relative to untreated roots. Data points from five biological replicates are plotted as open circles ( n ≥ 10). g – i Expression analysis of MtCLE13 and MtCEP7 genes in WT and nin mutant roots in response to a rhizobial inoculation 1 dpi ( g ), to an NF 10 −9 M treatment for 3 h ( h ), or to a cytokinin (BAP 10 −7 M) treatment for 3 h ( i ). qRT-PCR was used to measure the gene expression levels in treated roots, normalized relative to untreated roots. Data points from at least three biological replicates are plotted as open circles ( n = 8 except i , n ≥ 5). In a – i , center lines show the medians; box limits indicate the 25th and 75th percentiles as determined by the R software; whiskers extend 1.5 times the interquartile range from the 25th and 75th percentiles, outliers are represented by dots; and crosses represent sample means. Mann–Whitney test was used for each gene to assess significant differences between treatments in the WT and in the mutant (in a – c and g – i ) or between treated and control conditions (in d – f ), as indicated by asterisks (* α < 0.05; ** α < 0.01; *** α < 0.001). Full size image As the expression of MtNIN was previously shown to be induced by both NF and cytokinin treatments [9] , [11] , [12] and that MtCLE13 expression depends on MtNIN [46] , we analyzed the ability of MtNIN to regulate MtCLE13 and MtCEP7 expression. The results showed that the upregulation of MtNIN expression by rhizobia, NF, or cytokinin treatments was consistent with the rapid induction of MtCEP7 and MtCLE13 expression (Fig. 2d–f ), suggesting that these regulations might be mediated by MtNIN. By contrast, an analysis of MtCEP7 and MtCLE13 expression after a rhizobial, NF or cytokinin treatment in the nin mutant revealed that MtCLE13 and MtCEP7 gene induction was compromised (Fig. 2g–i ). Overall, these results indicate that the MtCRE1 cytokinin receptor and the MtNIN TF are required for the regulation of MtCLE13 and MtCEP7 expression by rhizobia, NFs, and cytokinins. MtCEP7 is induced in the root epidermis by rhizobium MtNIN and MtCLE13 genes were previously shown to be expressed in the epidermis as well as in the cortex of roots inoculated with rhizobia [15] , [25] , [28] , whereas the MtCEP7 expression pattern was never investigated. We used a pCEP7:GUS transcriptional fusion to determine the spatiotemporal expression of MtCEP7 . Uninoculated roots showed basal expression in the stele (Fig. 3a ), whereas the rhizobial inoculation rapidly induced pCEP7:GUS expression in epidermal cells within 4–24 h post inoculation (hpi; Fig. 3b–e ). At 4 dpi, MtCEP7 expression then followed the progression of rhizobial infections and was detected in nodule primordia (Fig. 3f–h ). In mature nodules, MtCEP7 expression was expressed in dividing cells at the nodule apex and in the vascular bundles (Supplementary Fig. 2A, B ). Concordantly, a quantitative reverse transcriptase polymerase chain reaction (qRT-PCR) analysis of the GUS transgene revealed the increased activity of the MtCEP7 promoter in roots inoculated with rhizobia (24 hpi and 4 dpi; Fig. 3i ). As anticipated from previous qRT-PCR analyses, the symbiotic expression of MtCEP7 in the root epidermis is detected in the WT but not in the nin mutant (Fig. 3j, k ). Fig. 3: MtCEP7 expression pattern in rhizobium-inoculated roots. a – h Expression pattern of a pCEP7:GUS transcriptional fusion. The GUS activity was analyzed in roots uninoculated ( a ) or inoculated with rhizobia 4 h post inoculation (hpi; b , c ), 24 hpi ( d , e ), 4 days post rhizobial inoculation (dpi; f , g ), or in a nodule primordium (5 dpi; h ). c is a detail of b , and g is a detail of f , as indicated by white squares. All images show longitudinal roots, except e that is a transversal section. All images show the GUS staining as a blue signal in bright field microscopy. The arrowhead in g indicates an infection thread. At least eight independent roots were analyzed for each condition from five independent experiments. Scale bars = 200 µm. i Expression analysis of GUS transcripts in pCEP7:GUS transgenic roots, assessed by qRT-PCR. Expression levels were normalized relative to uninoculated roots (0 hpi). To highlight fold changes, the dotted line corresponds to a ratio of 1. Center lines show the medians; box limits indicate the 25th and 75th percentiles as determined by the R software; whiskers extend 1.5 times the interquartile range from the 25th and 75th percentiles, outliers are represented by dots; crosses represent sample means; and data points from three biological replicates are plotted as open circles ( n = 9). Mann–Whitney test was used to assess significant differences between each time point and the non-treated control, as indicated by asterisks (*** α < 0.001). j , k Expression pattern of the pCEP7:GUS transcriptional fusion in WT ( j ) versus nin mutant roots 4 dpi ( k ). In a – h , j , k , a minimum of eight independent roots per experiment were analyzed for each time point, and five independent experiments were performed. Images show the GUS staining as a blue signal in bright field microscopy. Scale bars = 200 µm. Full size image MtNIN binds and transactivates MtCLE13 and MtCEP7 As NIN directly regulates CLE-RS genes in L. japonicus [32] , we tested whether such regulation was conserved in M. truncatula , and whether it could be shared for the regulation of the MtCEP7 gene. The analysis of MtCLE13 and MtCEP7 proximal promoters revealed the presence of a sequence similar to the NIN-binding site (NBS) previously described in L. japonicus (ref. [32] ; Fig. 4a, b ). We thus performed chromatin immunoprecipitation (ChIP) in rhizobia-inoculated roots of WT plants and nin mutants, with a native antibody targeting MtNIN previously validated in Vernié et al. [47] , or with immunoglobulin G (IgG) used as a negative control to evaluate non-specific binding. The IP enrichment of each promoter was measured by quantitative PCR (qPCR) using primers designed in the proximal regions of the MtCLE13 and MtCEP7 promoters that contained the predicted NBS cis -element identified, or in distal regions (Fig. 4b ). An enrichment of the proximal region of the MtCLE13 promoter was detected in the MtNIN IP, compared to the more distal region (Fig. 4c , left panel). This enrichment was not detected for MtNIN IPs performed in the nin mutant, as expected for a negative control. This result indicates a conservation of the NIN interaction with the promoter of a nodulation-related CLE peptide encoding gene between M. truncatula and L. japonicus . Furthermore, the MtNIN ChIP also revealed enrichment for the MtCEP7 proximal promoter region, relative either to the more distal promoter region or to the MtNIN IP performed in the nin mutant, as negative controls (Fig. 4c , right panel). This suggests that NIN co-regulates MtCLE13 and MtCEP7 expression. In order to determine whether MtNIN is sufficient to transactivate MtCLE13 and MtCEP7 gene expression, transient transformation assays were performed in M. truncatula mesophyll protoplasts (Fig. 4d ). To this aim, either a p35S:3xHA-NIN construct or the corresponding empty vector was co-transformed with a luciferase reporter gene driven either by the MtCLE13 or the MtCEP7 promoter region. After normalization of transfection efficiency with a pAtUbi:GUS control, the pMtCLE13:LUC and pMtCEP7:LUC activities were found as significantly enhanced by MtNIN ectopic expression (Fig. 4d ). These results indicate that MtNIN transactivates the expression of MtCLE13 and MtCEP7 . Fig. 4: NIN binds promoters and transactivates the expression of CLE13 and CEP7 . a Alignment of NIN-binding site (NBS) motifs previously identified in LjNF-YA1 , LjCLE-RS1 , and LjCLE-RS2 promoters [32] with homologous regions of MtNF-YA1 , MtCLE13 , and MtCEP7 promoters. Bold characters represent nucleotides conserved in more than four sequences out of the six identified. The sequence logo is derived from the six candidate NBSs, aligned using the MEME algorithm ( http://meme-suite.org/index.html ). b Schematic representation of MtCLE13 and MtCEP7 genes highlighting promoter regions used for ChIP-qPCR analyses. Red boxes represent the predicted NBSs identified on each promoter sequence. c NIN binds to the MtCLE13 and MtCEP7 promoters. Chromatin immunoprecipitation (ChIP)-qPCR analysis of NIN binding to MtCLE13 (left panel) and MtCEP7 (right panel) promoters, in wild-type (WT) or nin mutant roots 5 days post rhizobium inoculation (dpi) using either an anti-NIN antibody or IgG as a negative control. The fold enrichment of NIN binding was determined relative to IgG (control) IPs. One representative biological replicate out of two is shown. Data points from three technical replicates are plotted as open circles. d NIN transactivates MtCLE13 and MtCEP7 gene expression in M. truncatula mesophyll protoplasts. The promoter regions of MtCLE13 (left panel) and MtCEP7 (right panel) were fused to the luciferase (LUC) reporter gene and co-transformed in protoplasts with a p35S:NIN or an empty vector (ev). An AtUbi:GUS construct was used to measure the transformation efficiency. LUC/GUS ratios were normalized relative to values obtained in protoplasts transformed with an ev. To highlight fold changes, the dotted line corresponds to a ratio of 1. Data points from three biological replicates are plotted as open circles ( n = 6). Mann–Whitney test was used for each promoter to assess significant differences between LUC/GUS ratios in the presence or absence of the NIN construct, as indicated by asterisks (*** α < 0.001). e NIN activates MtCLE13 and MtCEP7 gene expression in M. truncatula roots. Expression analysis by qRT-PCR of MtNIN , MtCLE13 , and MtCEP7 in wild-type (WT) uninoculated roots transformed with a pAtUbi:NIN construct or an ev. Plants were grown on a nitrogen-free Fåhraeus medium. To highlight fold changes, expression levels were normalized relative to roots transformed with the ev. Data points from six biological replicates are plotted as open circles ( n ≥ 12). Mann–Whitney test was used for each gene to assess significant differences between pUbi:NIN-transformed roots and control roots, as indicated by asterisks (*** α < 0.001). f NIN expression driven by the pNIN 5kb promoter is sufficient to restore the regulation of MtCLE13 and MtCEP7 gene expression in response to rhizobium. nin mutant roots were transformed with either an ev or the pNIN 5kb :NIN construct. MtCLE13 and MtCEP7 gene expression was analyzed by qRT-PCR in roots grown in vitro on a nitrogen-free Fåhraeus medium, 2 dpi with rhizobium. Expression levels were normalized relative to uninoculated roots for each genotype. To highlight fold changes, the dotted line corresponds to a ratio of 1. Data points from five biological replicates are plotted as open circles ( n ≥ 9). Mann–Whitney test was used for each gene to assess significant differences between roots transformed with the pNIN 5kb :NIN construct and the control, as indicated by asterisks (*** α < 0.001). In c – f , center lines show the medians; box limits indicate the 25th and 75th percentiles as determined by the R software; whiskers extend 1.5 times the interquartile range from the 25th and 75th percentiles, outliers are represented by dots; and crosses represent sample means. Full size image To determine whether the ectopic expression of MtNIN could activate MtCEP7 and/or MtCLE13 expression in M. truncatula roots, MtNIN was constitutively expressed using the AtUbi promoter, and MtNIN , MtCLE13 , and MtCEP7 transcript levels were analyzed in uninoculated transformed roots (Fig. 4e ). In these conditions, the high expression level of MtNIN corresponds to the transgene ectopic expression, which was sufficient to increase the expression of both MtCLE13 and MtCEP7 genes. Accordingly, ectopic expression of MtNIN from the pUbi promoter was sufficient to induce the expression of the MtCEP7:GUS fusion in the absence of any symbiotic treatment, notably in the root epidermis (Fig. 5a–c ). The ectopic expression of MtNIN therefore bypasses the need for rhizobium, NF, or cytokinin treatments to induce MtCLE13 and MtCEP7 expression. Fig. 5: The NIN-binding site cis -element predicted in the proximal region of the CEP7 promoter is required for its induction by rhizobia. a – c NIN expression driven by the pUbi promoter is sufficient to induce the expression of a MtCEP7:GUS fusion in the absence of rhizobium ( b ), compared to an empty vector (ev) control ( a ). Representative images of the GUS expression pattern associated only with the root stele (“stele”) or with both the root epidermis and stele (“epidermis and stele”). Wild-type plants were grown in vitro on a nitrogen-free Fåhraeus medium. In c, quantification of the proportion of roots ( n ≥ 25) showing a GUS expression pattern associated only with the root stele or with both the root epidermis and stele, as described in a , b . d – h The NIN-binding site (NBS) in the proximal region of the MtCEP7 promoter is required for the induction of a MtCEP7:GUS fusion in response to rhizobium. In d , schematic representation of the MtCEP7 promoter, highlighting the predicted NBS cis -element identified as a red box and the corresponding deletion construct ( pCEP7ΔNBS:GUS ). In e , quantification of the proportion of roots ( n ≥ 34) showing a GUS expression pattern associated only with the root stele (“stele”) or with both the root epidermis and stele (“epidermis and stele”), as described in f – i . In f , g , representative images of the GUS expression pattern associated only with the root stele or with both the root epidermis and stele of pCEP7ΔNBS:GUS 1 day post rhizobium inoculation (dpi) in longitudinal ( f ) or transversal ( g ) sections. In h , i , representative images for the same GUS expression patterns for MtCEP7:GUS roots 1 dpi in longitudinal ( h ) or transversal ( i ) sections. In a , b , f – i , a minimum of eight independent roots were analyzed for each time point from three independent experiments. Images show the GUS staining as a blue signal in bright field microscopy. Scale bars = 100 µm. In c , e , Fisher exact test was performed to assess significant differences in the proportion of roots ( n ≥ 25) showing the different GUS expression patterns between the NIN overexpressing ( c ), or NBS-deleted MtCEP7:GUS ( e ) roots, and the control, as indicated by asterisks (*** α < 0.001). Full size image We next determined whether the MtNIN-dependent regulation of MtCEP7 relied on the putative NBS cis -element previously identified in the proximal region of the promoter. To this aim, we generated a version of the CEP7 promoter deleted from this NBS sequence and fused to the GUS reporter gene (Fig. 5d ). After a short-term rhizobial inoculation (1 dpi), the symbiotic induction of the pCEP7ΔNBS:GUS promoter was abolished (Fig. 5e, h, i ) compared to the WT promoter (Fig. 5e–g ), notably in the root epidermis. This indicates that the NBS cis -element identified is required for the symbiotic regulation of MtCEP7 expression. Finally, to establish a link between MtNIN epidermal expression and the symbiotic regulation of MtCEP7 , we used the recently characterized 5 kb NIN promoter region ( pNIN 5kb :NIN ) that is expressed in the root epidermis but not in the root cortex and that can specifically rescue the infection phenotype of the nin mutant [25] . This pNIN 5kb :NIN construct introduced in nin mutant roots was sufficient to restore expression of MtCEP7 as well as of MtCLE13 (Fig. 4f ). These results suggest that the MtNIN expression domain associated with the root epidermis is sufficient to induce both MtCEP7 and MtCLE13 expression in response to rhizobia. MtCEP7 peptides promote nodulation and rhizobial infections To evaluate the function of MtCEP7 peptides in early nodulation, exogenous treatments were first performed using peptide sequences corresponding to the conserved Domain 1 (MtCEP7 D1) or Domain 2 (MtCEP7 D2) regions (Fig. 6a , Supplementary Fig. 3A ). A similar enhancement of the number of nodules was observed compared to non-treated roots (Fig. 6b, c ). As effects on nodulation of another CEP peptide, MtCEP1, were previously shown to rely on the MtCRA2 CEP receptor homolog [39] , [41] , MtCEP7 peptides were thus exogenously applied on cra2 mutant roots. Positive effects on nodule number induced both by MtCEP7 D1 and D2 peptides relied on the MtCRA2 pathway (Fig. 6b, c ). Grafting experiments revealed that the activity of the MtCRA2 receptor was required in shoots to mediate the MtCEP7 positive effect on nodule number (Supplementary Fig. 4A ). In addition, split-root experiments were conducted where only half of the root system was treated with exogenous MtCEP7 peptides but nodule numbers quantified in parallel in locally treated roots and in distant non-treated (systemic) roots. This analysis revealed that the number of nodules was increased not only in MtCEP7-treated roots but also systemically in non-treated roots (Supplementary Fig. 4B ). Collectively, these results indicate that MtCEP7 regulates positively nodule number depending on the MtCRA2 receptor and that this regulation occurs systemically in the root system thanks to the action of MtCRA2 in shoots. Fig. 6: CEP7 peptides regulate positively nodule number and rhizobial infections. a Schematic representation of the predicted MtCEP7 prepropeptide. The blue rectangle represents the N-terminal signal peptide predicted using SignalP 3.0 ( http://www.cbs.dtu.dk/services/SignalP-3.0/ ). Red rectangles represent the predicted MtCEP7 Domain 1 (CEP7 D1) and Domain 2 (CEP7 D2) peptide sequences with hydroxyl modifications to proline as indicated in bold. b Representative images of the nodulation phenotype of wild-type (WT) and cra2 mutants treated with synthetic CEP7 D1 or CEP7 D2. Scale bars = 1 cm. c Quantification of the nodule number in WT and cra2 mutants, grown in vitro on a nitrogen-free Fåhraeus medium supplemented or not with 1 µM CEP7 D1 or CEP7 D2 peptides. Nodule number was scored at 14 days post rhizobium inoculation (dpi). Graphs are based on data points from three biological replicates ( n ≥ 59). Mann–Whitney test was used for each genotype to assess significant differences between peptide-treated and control plants, as indicated by asterisks (*** α < 0.001). d The nodulation phenotype of plants expressing an artificial microRNA targeting MtCEP7 transcripts (amiRCEP7). Representative images of nodulated roots transformed either with an empty vector (ev) or with the amiRCEP7 construct described in d . Scale bars = 1 cm. e Quantification of the nodule number of plants transformed either with an ev or with an amiRCEP7 construct. Plants were grown in vitro on a nitrogen-free Fåhraeus medium and nodules were scored at 14 dpi. Graphs are based on data points from 1 representative biological replicate out of 3 ( n ≥ 14). Mann–Whitney test was used to assess significant differences, as indicated by asterisks (* α < 0.05). f Quantification of infection thread (IT) number in six dpi roots transformed either with an ev or with the amiRCEP7 construct and inoculated with a rhizobium strain constitutively expressing a LacZ reporter. ITs that reached the epidermis (epidermal ITs) were distinguished from ITs that reached the cortex (cortical ITs). Graphs are based on data points from two biological replicates ( n ≥ 15). Mann–Whitney test was used to assess significant differences between amiRCEP7 roots and control roots, as indicated by asterisks (* α < 0.05; *** α < 0.001). g Representative images of the nodulation phenotype of plants transformed either with a pCLE13:GUS or a pCLE13:CEP7 construct. Scale bars = 1 cm. h Quantification of the nodule number in plants transformed either with the pCLE13:CEP7 construct or the pCLE13:GUS construct as a negative control. Plants were grown in pots containing a perlite/sand (3/1) mixture and watered with a “i” low nitrogen medium, and nodules were scored at 21 dpi. Graphs are based on data points from two biological replicates ( n ≥ 28). Mann–Whitney test was used to assess significant differences, as indicated by asterisks (** α < 0.01). i Quantification of IT number in six dpi roots transformed either with the pCLE13:CEP7 construct or the pCLE13:GUS construct as a negative control and inoculated with a rhizobium strain constitutively expressing a LacZ reporter. ITs that reached the epidermis (epidermal ITs) were distinguished from ITs that reached the cortex (cortical ITs). Graphs are based on data points from two biological replicates ( n ≥ 15). Mann–Whitney test was used to assess significant differences between the pCLE13:CEP7 roots and control roots, as indicated by asterisks (** α < 0.01; *** α < 0.001). In c , e , f , h , i , center lines show the medians; box limits indicate the 25th and 75th percentiles as determined by the R software; whiskers extend 1.5 times the interquartile range from the 25th and 75th percentiles, outliers are represented by dots; and crosses represent sample means. Full size image To independently validate the function of MtCEP7 in early nodulation, loss-of-function approaches were additionally performed. Two independent strategies were used, namely, the silencing of MtCEP7 expression by an RNAi ( MtCEP7 RNAi) or by an artificial microRNA (amiRNA) approach (amiRCEP7; regions targeted by each construct are shown in Supplementary Fig. 3B ). The number of nodules of MtCEP7 RNAi roots was lower than for GUS RNAi control roots (Supplementary Fig. 5A ), which agrees with results of the previous exogenous peptide treatments. Similarly, amiRCEP7 roots formed a reduced number of nodules compared to control roots (Fig. 6d, e ). The strength of nodule number phenotypes was correlated to the efficiency and specificity of these approaches, evaluated by qRT-PCR on the different CEP peptide-encoding genes (Supplementary Fig. 5B, C ). Collectively, these results suggest that the MtCEP7 peptide has a positive role in nodulation but that a redundant function with other CEP peptide-encoding genes likely exists. Since MtNIN expression in the root epidermis restores the symbiotic induction of MtCEP7 expression (Fig. 4f ), the role of MtCEP7 peptides in the regulation of rhizobial infections was further investigated using the amiRCEP7 construct shown previously to affect more strongly nodule number. To this aim, we used a Sinorhizobium strain expressing constitutively a LacZ marker to visualize infection events in roots (Fig. 6f ). The number of ITs was reduced in roots expressing the amiRCEP7 construct relative to control roots, mostly in the root epidermis. As an independent validation, a stable line expressing the pENOD11-GUS symbiotic infection marker was used (Supplementary Fig. 6 ). The number of MtENOD11 -positive infection foci was similarly significantly reduced in amiRCEP7 roots, mostly in epidermal cells but also in cortical cells (Supplementary Fig. 6A, B ). Collectively, these results indicate that the MtNIN-dependent induction of MtCEP7 expression positively regulates rhizobial infections. To evaluate the functional relevance of the symbiotic activation of MtCEP7, we used the MtCLE13 promoter to ectopically express MtCEP7 in the same spatiotemporal symbiotic domain as this negatively acting CLE peptide [28] , [36] . The MtCEP7 expression level increased ~35-fold in pCLE13 : MtCEP7 roots compared to p CLE13:GUS control roots (Supplementary Fig. 5D ) and was associated with a significant increase in the number of nodules formed on p CLE13:CEP7 roots relative to control roots (Fig. 6g, h ). In addition, the number of ITs was evaluated, using the LacZ-expressing Sinorhizobium strain (Fig. 6i ), revealing a significant increase in p CLE13:CEP7 roots relative to control roots both in the epidermis and in the cortex. Overall, these results suggest that increasing the level of MtCEP7 activity may mitigate the CLE13-dependent negative AON regulation of nodule number and symbiotic infections. In this study, we show that the MtCEP7 gene is rapidly upregulated by rhizobia as well as by NFs and cytokinins, suggesting that MtCEP7 may have a function more specifically related to symbiotic nodulation. A combination of gain-of-function experiments, based on exogenous treatment applications and ectopic expression, as well as of loss-of-function experiments, based on RNAi and amiRNA strategies, support a positive function of MtCEP7 in promoting nodulation and rhizobial infections. The previously observed increased nodulation induced by the ectopic expression of MtCEP1 or by the addition of MtCEP1 peptides mimics the effect of MtCEP7 [3] , [38] , [40] , even though a MtCEP1 knock-down affecting also MtCEP2 expression does not alter nodulation, despite promoting lateral root formation and thus indicating the efficiency of the RNAi approach [38] . Among all other CEP-encoding genes, the unique feature of the MtCEP7 gene to be induced by rhizobia supports a role in maintaining a window for new nodule formation after the initial rhizobial infections occurred. Given that legume symbiotic nodulation emerged during evolution after the emergence of CEP [48] and CLE genes [49] , the identification of a NF-dependent symbiotic expression pattern for MtCEP7 , or MtCLE12 and MtCLE13 , suggests a sub-functionalization of these genes within their respective families. The loss-of-function approaches, however, highlight the possibility that a functional redundancy of MtCEP7 likely exist with other CEP encoding gene(s) that is (are) not upregulated rapidly after Sinorhizobium meliloti inoculation. The fast induction of MtCEP7 expression in response to rhizobia led us to analyze its regulation in response to NF signals. In agreement with RNAseq datasets from Jardinaud et al. [15] showing an NF induction of MtCEP7 in the root epidermis, we now show that rhizobia also rapidly induces the expression of this gene in a subset of root epidermal cells. This expression then follows the progression of rhizobial infections to finally reach the growing nodule primordium. Since the MtCRA2 and MtSUNN receptors are not expressed in the root epidermis either with or without NF [15] , the symbiotically induced expression of MtCEP7 and MtCLE13 likely acts non-cell autonomously. Previous work indicated that MtCEP1 phenotypes relied on the activity in shoots of the CRA2 receptor [39] , [41] , which appears functionally orthologous to the CEPR1 CEP receptor of Arabidopsis [3] , [43] , [50] . Similarly, we now show using both hypocotyl grafts between the WT and the cra2 mutant and split-root experiments with CEP7 peptides that the promotion of nodulation induced by MtCEP7 peptides relies on MtCRA2 and that this regulation occurs systemically in distant non-treated roots through the activity of the MtCRA2 receptor in shoots. There is scarce knowledge on how peptide hormone signaling intersects with metabolite hormones, such as cytokinin [51] , [52] . An example in Arabidopsis is the regulation by WUSCHEL of AtCLV3 expression in the shoot apical meristem, which is itself a direct target of cytokinin signaling [52] , [53] . The M. truncatula model offers a unique opportunity to dissect how two independent systemic signaling pathways regulate symbiotic nodulation antagonistically [36] , [41] . To our knowledge, we show here for the first time in plants that a single TF, MtNIN, which is upregulated by cytokinin, co-regulates the expression of two signaling peptides encoding genes from different families, MtCEP7 and MtCLE13 . Previously, MtCRE1 and MtNIN were shown to be required for the induction of MtCLE13 in response to cytokinin [28] , [46] . We now show that MtCRE1 and MtNIN also are required for the induction of MtCLE13 by NFs and rhizobia. This suggests that the direct regulation of AON-related CLE genes by NIN is evolutionary conserved between L. japonicus and M. truncatula (ref. [32] ; this study). Indeed, MtCLE13 expression is transactivated by MtNIN in a leaf mesophyll protoplast assay, its promoter bound by MtNIN in a ChIP-qPCR assay, and the ectopic induction of MtNIN in M. truncatula roots is sufficient to induce MtCLE13 expression. Strikingly, the same set of approaches revealed that MtNIN similarly binds the MtCEP7 promoter and transactivates its expression. As reported in L. japonicus [32] , a conserved NBS cis -element was identified in the MtCLE13 proximal promoter that corresponded to the NIN IP-enriched promoter region. Interestingly, an NBS cis -element was also identified in the NIN IP-enriched region of the MtCEP7 proximal promoter, which is required for its short-term regulation by rhizobia in the root epidermis. Our results also suggest that MtNIN regulates the expression of CLE13 and CEP7 in the same expression domain notably including the root epidermis. The identification of this MtNIN-mediated co-regulation opens perspectives to extrapolate this type of co-regulation for other nutritional contexts and in non-legume plants. It could be surprising that, at about the same time during early nodulation, MtNIN upregulates two signaling peptides that antagonistically regulate nodule number. It has to be noted, however, that the strength of the induction of MtCEP7 expression by rhizobia is different than for MtCLE13 [28] . This suggests that other TFs may be differentially recruited in addition to MtNIN to regulate MtCLE13 versus MtCEP7 expression. We used this differential symbiotic induction pattern to explore a potential functional relevance of this simultaneous induction of antagonistic nodulation-related signaling peptides by expressing MtCEP7 with the MtCLE13 promoter. Interestingly, an increased number of nodules was observed, suggesting that enhancing MtCEP7 in the MtCLE13 expression domain was able to mitigate the onset of the negative AON pathway. We thus speculate that the modulation of MtCEP7 and MtCLE13 expression through the rhizobium-/NF- and cytokinin-induced MtCRE1- and MtNIN-dependent signaling pathway may enable a dynamic fine-tuning of nodule number depending on plant’s metabolic capacities and needs. An attractive hypothesis is that the MtCEP7 pathway may be required to modulate the negative AON pathway during the plant life cycle, i.e., depending on growth needs that, for example, are driven by the shoot photosynthetic capacity. This implies that shoot-derived carbon signals may impact the MtCEP7 and MtCLE13 pathways, as recently shown in Arabidopsis for CEP genes [44] . In addition, an inhibitor of NIN function acting during early nodulation was identified recently in G. max , Nodule Number Control 1 (NNC1), which encodes an Apetala2-type TF that notably inhibits the NIN-dependent regulation of AON CLE peptide-encoding genes [31] . Further work is needed to determine whether this negative regulatory module is also recruited to modulate MtCEP7 expression. In the future, we also need to better understand which molecular mechanisms allow environmental conditions or the plant metabolic status to impact the balance between CLE-dependent negative and CEP-dependent positive systemic pathways that fine tunes nodule number and the number of infection events. Biological material, growth conditions, and treatments The M. truncatula Jemalong A17 WT genotype, as well as the cre1-1 , nin-1 , nfp-C31 , and cra2-11 mutants were used in this study. These mutants are described in Plet et al. [11] , Marsh et al. [23] , Ben Amor et al. [45] , and Laffont et al. [41] , respectively. The pENOD11:GUS transgenic line was generated in Journet et al. [7] . Seeds were scarified in sulfuric acid (Sigma, www.sigmaaldrich.com ) for 3 min, washed four times with distilled water, and then sterilized for 20 min in bleach (12% [v/v] sodium hypochlorite; Chlorifix, Bayrol, https://www.bayrol.fr/ ). After washings with sterile water, the seeds were placed on 1.5% water–agar plates (Bactoagar, Becton Dickinson), stratified for 2 days in the dark at 4 °C, and then germinated overnight at 24 °C. The germinated seedlings were grown in vitro vertically on square plates in a growth chamber at 24 °C under a long day photoperiod (16 h light; 150 μE intensity) on nitrogen-free Fåhraeus medium [54] . Alternatively, germinated seedlings were grown in pots containing a perlite:sand 3:1 mixture in a growth chamber (24 °C, 16 h light, 150 µmol m −2 s −1 ; relative humidity 60%) and watered every 2 days with the “i” low nitrogen medium (0.25 mM KNO 3 ) [55] . For nodulation experiments, the S. meliloti 1021 strain was used for in vitro experiments or the Sinorhizobium medicae WSM419 strain for plants grown in perlite/sand pots. To quantify infection events, a S. meliloti strain Sm 1021 carrying a pXLGD4 plasmid expressing a Pro HemA :LacZ marker (GMI6526; [56] ) was used to follow bacteria progression from root hairs to cortical cells. Five dpi roots were stained using a β-galactosidase histochemical assay as described in Ardourel et al. [56] and observed using a stereomicroscope (Olympus, BX53, www.olympus-lifescience.com/ ). In all cases, rhizobial strains were grown at 28 °C on a Yeast Extract Broth medium (YEB; Vervliet et al. [57] ) supplemented with streptomycin 50 mg L −1 for Sm 1021 or chloramphenicol 25 mg L −1 for WSM419, and plants were inoculated with an OD 600nm = 0.05 bacterial suspension. For the nodulation kinetic experiments, roots or developing nodules from at least eight individual plants per biological replicate were harvested 0, 1, 4, 8, and 14 dpi and frozen in liquid nitrogen for further RNA extraction. For cytokinin and NF treatments, about 25 germinated seedlings were grown on a grid in a Magenta box filled with “i” low nitrogen liquid medium, under gentle agitation at 24 °C and with a long day photoperiod (24 °C, 16 h light, 150 µmol m −2 s −1 ). After 6 days, seedlings were treated or not with the cytokinin BAP 10 −7 M (Sigma-Aldrich), or with NF 10 −9 M, and grown under the same conditions. Treated or untreated roots (mock) from at least 10 individual plants per biological replicate were harvested after 3 h and immediately frozen in liquid nitrogen prior to RNA extraction. For peptide treatments, about 25 germinated seedlings were grown on nitrogen-free Fåhraeus medium with or without 1 µM synthetic peptides corresponding to the conserved domains of MtCEP7 (GL Biochem Ltd, China): MtCEP7 Domain 1 (CEP7 D1), SFRhyPTTPGSShyPGVGH; and MtCEP7 Domain 2 (CEP7 D2), GFKhyPTNPSHShyPGVGH (where “hyP” indicates proline hydroxylation). Plants were grown in a growth chamber (22 °C, 16 h light, 100 µmol m −2 s −1 ). Grafts were generated in vitro as described in the “Medicago handbook” ( http://www.noble.org/medicagohandbook/ ) or according to the hypocotyl grafting technique described in Chapman et al. [50] and then transferred after 2 weeks on nitrogen-free Fåhraeus medium with or without 1 µM synthetic MtCEP7 D1 peptides in the same growth conditions as previously described. Grafts were inoculated 1 week after transfer, and the nodule number was scored 7 and 14 days post Sinorhizobium inoculation. Split roots were generated in vitro using Fåhraeus medium supplemented with 5 mM KNO 3 . Seedlings were grown for 24 h and root tips were cut and then grown for 4 days under the growth conditions previously described. Plants with two equivalent roots were then selected and transferred onto a nitrogen-free Fåhraeus medium where the agar was split. CEP7 D1 synthetic peptide (1 µM) was added, or not, to one half of the agar plate before the plants were transferred. Split roots were inoculated with rhizobia 3 days after transfer, and the nodule number was scored at 14 dpi in treated and untreated roots. Cloning and Agrobacterium rhizogenes root transformation Using the Gateway technology, an RNAi construct targeting the MtCEP7 gene was generated by PCR amplification of a 250-nt MtCEP7 region (indicated by nucleotides in blue in Supplementary Fig. 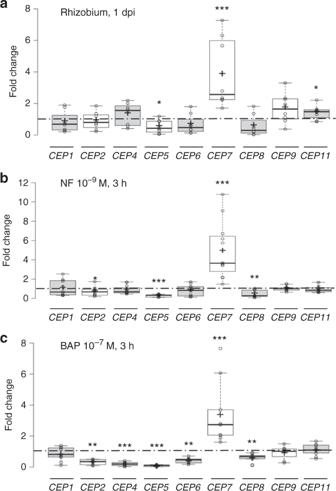Fig. 1: Expression of CEP peptide-encoding genes in response to rhizobia, Nod factors, or cytokinins. aExpression analysis ofCEPgenes in wild-type (WT) roots 1 day post rhizobial inoculation (1 dpi). qRT-PCR was used to measure theCEPgene expression levels, normalized relative to uninoculated roots. To highlight fold changes, the dotted line corresponds to a ratio of 1. Data points from four biological replicates are plotted as open circles (n= 8).bExpression analysis ofCEPgenes in WT roots in response to a Nod factor (NF) 10−9M treatment for 3 h. qRT-PCR was used to measure theCEPexpression levels in treated roots. The results were normalized relative to untreated roots. To highlight fold changes, the dotted line corresponds to a ratio of 1. Data points from six biological replicates are plotted as open circles (n≥ 11).cExpression analysis ofCEPgenes in WT roots in response to a cytokinin (BAP 10−7M) treatment for 3 h. qRT-PCR was used to measure theCEPgene expression levels in treated roots. The results were normalized relative to untreated roots. To highlight fold changes, the dotted line corresponds to a ratio of 1. Data points from four biological replicates are plotted as open circles (n≥ 8). Ina–c, center lines show the medians; box limits indicate the 25th and 75th percentiles as determined by the R software; whiskers extend 1.5 times the interquartile range from the 25th and 75th percentiles, outliers are represented by dots; and crosses represent sample means. Mann–Whitney test was used for each gene to assess significant differences between treated and control conditions, as indicated by asterisks (*α< 0.05; **α< 0.01; ***α< 0.001). 2 ) using primers flanked with attB recombination sites (primers listed in Supplementary Table 1 ), which was inserted into the pDONR221 vector (ThermoFisher, www.thermofisher.com ), subsequently recombined into the pFRN binary vector [9] , and then validated by sequencing. The pFRN GUS RNAi kanamycin-resistant vector previously described in Gonzalez-Rizzo et al. [9] was used as a control. The efficiency of the MtCEP7 RNAi construct was evaluated on roots collected 2 days post rhizobia inoculation (dpi), immediately frozen in liquid nitrogen for further RNA extraction. For the CEP7 promoter transcriptional fusion with GUS , a 2-kb region upstream of the predicted ATG was selected and amplified from genomic Jemalong A17 DNA, cloned into pENTR/D TOPO (ThermoFisher, http://www.thermofisher.com ), sequenced, and subsequently transferred into the pKGWFS7 destination vector (spectinomycin/streptinomycin resistance for bacterial selection; ref. [58] ). The p35S:3xHA-NIN construct (carbenicillin resistant) was previously generated in Vernié et al. [47] , whereas the pNIN 5kb :NIN construct and the corresponding empty vector (spectinomycin resistant) were generated in Liu et al. [25] . Other constructs were generated using a Golden Gate strategy, as described in Engler and Marillonnet [59] , with vectors generated by Weber et al. [60] and provided by the Engineering Nitrogen Symbiosis for Africa (ENSA) project ( https://www.ensa.ac.uk/ ). For protoplast transformation, pCEP7:LUC , pCLE13:LUC , and pAtUbi:GUS single gene constructs (promoter–gene–terminator) were cloned into a level 1 Golden Gate vector (EC47811, ampicillin resistant). For M. truncatula root transformation , pAtUbi:amiRCEP7 , pCLE13:CEP7 , pCLE13:GUS , pCEP7:GUS and pAtUbi:NIN:GFP constructs were first cloned into the level 1 vector (EC47811), which was then combined with a pNOS:Kanamycin cassette (EC15029), to allow in planta kanamycin selection of transformed roots into a level 2 destination vector (EC50507). For co-expression experiments, pCEP7:GUS and pAtUbi:NIN:GFP constructs were combined into a single vector. LUC (EC15217), GUS (EC75111), GFP (EC15095), pAtUbi (EC15062), and 35S terminator (EC41414) cassettes were also provided by the ENSA project. For the CEP7 promoter, a ~2.4-kb region upstream of the predicted ATG was selected, whereas the ~2-kb region of the MtCLE13 promoter previously characterized by Mortier et al. [28] was used and amplified by PCR on Jemalong A17 genomic DNA using primers listed in Supplementary Table 1 . The same region of the MtCLE13 promoter was used to express MtCEP7 using the level 1 vector. The efficiency of this MtCEP7 ectopic expression construct was evaluated on roots collected 21 dpi. The pCEP7ΔNBS:GUS promoter was constructed by combining two PCR products, amplified, respectively, right upstream and downstream of the predicted NBS cis -element (primers listed in the Supplementary Table 1 ). The pAtUbi:amiRCEP7 amiRNA construct was designed based on the Carbonell et al. [61] strategy (amiRNA sequence provided in Supplementary Table 1 ). The amiRCEP7 cassette was synthetized by Genewiz ( https://www.genewiz.com/ ) and then assembled with the pAtUbi promoter in the level 1 vector. The efficiency of the amiRCEP7 construct was evaluated on roots collected 2 dpi. Constructs of interest were then introduced into the A. rhizogenes ARqua1 strain and recombinant Arqua1 bacteria were used to transform roots according to the protocol described in Boisson-Dernier et al. [62] . The A. rhizogenes strains were grown at 28 °C for 2 days on a YEB-agar medium supplemented with appropriate antibiotics (Duchefa, https://www.duchefa-biochemie.com/ ). Infected seedlings were grown in vitro on a Fåhraeus medium supplemented with 1 mM NH 4 NO 3 (Truchet et al.) [54] and kanamycin (25 mg L −1 ; Duchefa) for 1 week at 20 °C, and 1 more week at 24 °C under a 16-h light photoperiod (150 μE). Plantlets with kanamycin-resistant transformed roots were then transferred either in vitro onto a growth paper (Mega International, http://www.mega-international.com/ ) on nitrogen-free Fåhraeus medium, grown for 5 days, and then inoculated with rhizobia as previously described or transferred to pots containing a perlite:sand 3:1 mixture for 5 days and then inoculated with rhizobia. Nodule number was scored at 14 dpi for plants grown in vitro or at 21 dpi for plants grown in perlite/sand pots. Images of nodules were obtained in bright field using an AxioZoom V16 macroscope (Zeiss, https://www.zeiss.fr ). Transient activation assays in M. truncatula protoplasts Leaf protoplasts were isolated from 8-week-old M. truncatula plants as described by Yoo et al. [63] , except that 2% Cellulase Onozuka R10 (Yakult Pharmaceutical Industry CO LTD), 1% Macerozyme R10 (Yakult Pharmaceutical Industry CO LTD), and 4% Viscozyme (Sigma) enzymes were used to digest the cell walls. Protoplasts (2.5 × 10 5 ) were transfected with 20 μg of a DNA mixture consisting of 9 μg of either the pCLE13:LUC or the pCEP7:LUC reporter construct, 10 µg of the p35S-3xHA-NIN or of the empty vector construct as a negative control, and 1 μg of the pAtUbi:GUS vector used as an internal control to normalize the transfection efficiency. After transfection, the protoplasts were incubated overnight at 20 °C in darkness. Protoplasts were then harvested by centrifugation (100 × g for 5 min), lysed in a protoplast lysis buffer [63] , and protein extracts were clarified by centrifugation (2000 × g for 5 min). For GUS assays, protein extracts were incubated 30 min at 37 °C with the 4-methylumbelliferyl-β- d -glucuronide hydrate (MUG, Duchefa, https://www.duchefa-biochemie.com/ ) substrate (1 mM 4-MUG in 50 mM sodium phosphate (pH 7.0), 0.1% Triton X-100, 10 mM EDTA, 0.1% sodium lauryl sarcosine, and 10 mM dithiothreitol (DTT)), and fluorescence was measured with an Infinite200 microplate reader (Tecan, http://www.tecan.com ). For luciferase (LUC) assays, protein extracts were mixed with a luciferase assay buffer (20 mM Tricine pH 7.8, 5 mM MgCl2, 0.1 mM EDTA, 3.3 mM DTT, 270 µM Coenzyme A, 500 µM Luciferin (Duchefa), and 500 µM ATP), and luminescence was immediately measured for 10 s using the Tecan Infinite200 microplate reader. 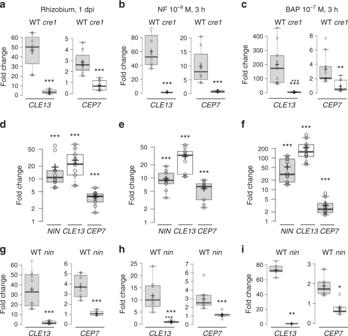Fig. 2: Rhizobia, Nod factor, and cytokinin regulation ofCEP7andCLE13expression relies on the CRE1 cytokinin receptor and on the NIN transcription factor. a–cExpression analysis of theMtCEP7andMtCLE13genes in wild-type (WT) orcre1mutant roots in response to a 1 day post rhizobial inoculation (1 dpi) (a), to a Nod factor (NF) 10−9M treatment for 3 h (b), or to a cytokinin (BAP 10−7M) treatment for 3 h (c). qRT-PCR was used to measure the gene expression levels in treated roots, normalized relative to untreated roots. Data points from four biological replicates are plotted as open circles (n≥ 8).d–fExpression analysis ofMtNIN,MtCLE13, andMtCEP7genes in WT roots in response to a rhizobial inoculation 1 dpi (d), to an NF 10−9M treatment for 3 h (e), or to a cytokinin (BAP 10−7M) treatment for 3 h (f). qRT-PCR was used to measure the gene expression levels in treated roots, normalized relative to untreated roots. Data points from five biological replicates are plotted as open circles (n≥ 10).g–iExpression analysis ofMtCLE13andMtCEP7genes in WT andninmutant roots in response to a rhizobial inoculation 1 dpi (g), to an NF 10−9M treatment for 3 h (h), or to a cytokinin (BAP 10−7M) treatment for 3 h (i). qRT-PCR was used to measure the gene expression levels in treated roots, normalized relative to untreated roots. Data points from at least three biological replicates are plotted as open circles (n= 8 excepti,n≥ 5). Ina–i, center lines show the medians; box limits indicate the 25th and 75th percentiles as determined by the R software; whiskers extend 1.5 times the interquartile range from the 25th and 75th percentiles, outliers are represented by dots; and crosses represent sample means. Mann–Whitney test was used for each gene to assess significant differences between treatments in the WT and in the mutant (ina–candg–i) or between treated and control conditions (ind–f), as indicated by asterisks (*α< 0.05; **α< 0.01; ***α< 0.001). LUC/GUS ratios were calculated and normalized relative to the empty vector. 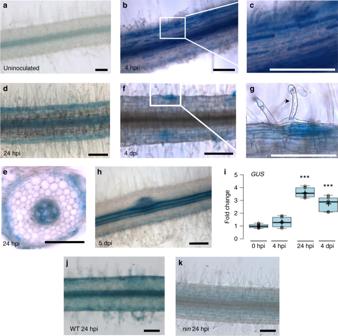Fig. 3:MtCEP7expression pattern in rhizobium-inoculated roots. a–hExpression pattern of apCEP7:GUStranscriptional fusion. The GUS activity was analyzed in roots uninoculated (a) or inoculated with rhizobia 4 h post inoculation (hpi;b,c), 24 hpi (d,e), 4 days post rhizobial inoculation (dpi;f,g), or in a nodule primordium (5 dpi;h).cis a detail ofb, andgis a detail off, as indicated by white squares. All images show longitudinal roots, except e that is a transversal section. All images show the GUS staining as a blue signal in bright field microscopy. The arrowhead ingindicates an infection thread. At least eight independent roots were analyzed for each condition from five independent experiments. Scale bars = 200 µm.iExpression analysis ofGUStranscripts inpCEP7:GUStransgenic roots, assessed by qRT-PCR. Expression levels were normalized relative to uninoculated roots (0 hpi). To highlight fold changes, the dotted line corresponds to a ratio of 1. Center lines show the medians; box limits indicate the 25th and 75th percentiles as determined by the R software; whiskers extend 1.5 times the interquartile range from the 25th and 75th percentiles, outliers are represented by dots; crosses represent sample means; and data points from three biological replicates are plotted as open circles (n= 9). Mann–Whitney test was used to assess significant differences between each time point and the non-treated control, as indicated by asterisks (***α< 0.001).j,kExpression pattern of thepCEP7:GUStranscriptional fusion in WT (j) versusninmutant roots 4 dpi (k). Ina–h,j,k, a minimum of eight independent roots per experiment were analyzed for each time point, and five independent experiments were performed. Images show the GUS staining as a blue signal in bright field microscopy. Scale bars = 200 µm. qRT-PCR gene expression analysis Total RNAs were isolated from frozen roots with the RNeasy Plant Mini Kit (Qiagen, http://www.qiagen.com/ ) according to the manufacturer’s instructions. 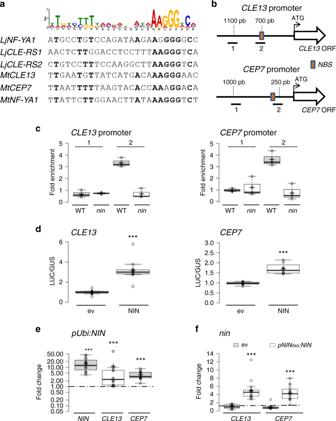Fig. 4: NIN binds promoters and transactivates the expression ofCLE13andCEP7. aAlignment of NIN-binding site (NBS) motifs previously identified inLjNF-YA1,LjCLE-RS1, andLjCLE-RS2promoters32with homologous regions ofMtNF-YA1,MtCLE13, andMtCEP7promoters. Bold characters represent nucleotides conserved in more than four sequences out of the six identified. The sequence logo is derived from the six candidate NBSs, aligned using the MEME algorithm (http://meme-suite.org/index.html).bSchematic representation ofMtCLE13andMtCEP7genes highlighting promoter regions used for ChIP-qPCR analyses. Red boxes represent the predicted NBSs identified on each promoter sequence.cNIN binds to theMtCLE13andMtCEP7promoters. Chromatin immunoprecipitation (ChIP)-qPCR analysis of NIN binding toMtCLE13(left panel) andMtCEP7(right panel) promoters, in wild-type (WT) orninmutant roots 5 days post rhizobium inoculation (dpi) using either an anti-NIN antibody or IgG as a negative control. The fold enrichment of NIN binding was determined relative to IgG (control) IPs. One representative biological replicate out of two is shown. Data points from three technical replicates are plotted as open circles.dNIN transactivatesMtCLE13andMtCEP7gene expression inM. truncatulamesophyll protoplasts. The promoter regions ofMtCLE13(left panel) andMtCEP7(right panel) were fused to the luciferase (LUC) reporter gene and co-transformed in protoplasts with a p35S:NIN or an empty vector (ev). An AtUbi:GUS construct was used to measure the transformation efficiency. LUC/GUS ratios were normalized relative to values obtained in protoplasts transformed with an ev. To highlight fold changes, the dotted line corresponds to a ratio of 1. Data points from three biological replicates are plotted as open circles (n= 6). Mann–Whitney test was used for each promoter to assess significant differences between LUC/GUS ratios in the presence or absence of the NIN construct, as indicated by asterisks (***α< 0.001).eNIN activatesMtCLE13andMtCEP7gene expression inM. truncatularoots. Expression analysis by qRT-PCR ofMtNIN,MtCLE13, andMtCEP7in wild-type (WT) uninoculated roots transformed with a pAtUbi:NIN construct or an ev. Plants were grown on a nitrogen-free Fåhraeus medium. To highlight fold changes, expression levels were normalized relative to roots transformed with the ev. Data points from six biological replicates are plotted as open circles (n≥ 12). Mann–Whitney test was used for each gene to assess significant differences between pUbi:NIN-transformed roots and control roots, as indicated by asterisks (***α< 0.001).fNINexpression driven by thepNIN5kbpromoter is sufficient to restore the regulation ofMtCLE13andMtCEP7gene expression in response to rhizobium.ninmutant roots were transformed with either an ev or thepNIN5kb:NINconstruct.MtCLE13andMtCEP7gene expression was analyzed by qRT-PCR in roots grown in vitro on a nitrogen-free Fåhraeus medium, 2 dpi with rhizobium. Expression levels were normalized relative to uninoculated roots for each genotype. To highlight fold changes, the dotted line corresponds to a ratio of 1. Data points from five biological replicates are plotted as open circles (n≥ 9). Mann–Whitney test was used for each gene to assess significant differences between roots transformed with thepNIN5kb:NINconstruct and the control, as indicated by asterisks (***α< 0.001). Inc–f, center lines show the medians; box limits indicate the 25th and 75th percentiles as determined by the R software; whiskers extend 1.5 times the interquartile range from the 25th and 75th percentiles, outliers are represented by dots; and crosses represent sample means. Total RNAs (1.5 µg) were used for cDNA synthesis with the Superscript II Reverse Transcriptase (ThermoFisher, http://www.thermofisher.com ). qRT-PCR experiments were performed on a LightCycler 480 apparatus using the LightCycler480 SYBR Green I Master Kit (Roche Diagnostics, http://lifescience.roche.com ) according to the manufacturer’s instructions. Cycling conditions were as follows: 95 °C for 5 min, and then 40 cycles at 95 °C for 15 s, 60 °C for 15 s, and 72 °C for 15 s. A dissociation curve (55–95 °C) was performed to assess the specificity of the amplification. The expression of genes of interest was normalized against the reference genes MtACTIN11 and MtRBP1 ( RNA binding protein 1 ) previously selected using the Genorm software ( https://genorm.cmgg.be/ ) [64] . All primers used in qRT-PCR are listed in Supplementary Table 1 . Cycle threshold (Ct) values obtained for the two reference genes were averaged prior to calculation of ratios of genes of interest onto reference genes. These ratios were calibrated relative to the experimental control condition (WT genotype and/or untreated mock control). ChIP-qPCR assays ChIP experiments were performed on WT or nin roots (~3 g of fresh weight) grown in vitro on a nitrogen-free Fåhraeus medium and inoculated 5 days with rhizobia. Briefly, after plant material fixation in 1% (v/v) formaldehyde for 30 min, roots were frozen and ground in liquid nitrogen; then nuclei were isolated and lysed according to Gendrel et al. [65] . Chromatin was then sonicated using a water bath Bioruptor® Plus sonicator (Diagenode; 40 cycles of 30 s on/30 s off pulses). IPs were performed on the sonicated chromatin using an α-NIN antibody (5:1000; Vernié et al. [47] ) or IgG (Sigma Aldrich) as a negative control, as described in Gendrel et al. [65] , except that washes were performed with a lower stringency using a ChIP dilution buffer (167 mM NaCl, 16.7 mM Tris-Hcl pH 8, 1.2 mM EDTA, 1.1% Triton X-100). Immunoprecipitated DNA was analyzed by qPCR (Roche Diagnostics, http://lifescience.roche.com ) as previously described for RT-PCR, using primers listed in Supplementary Table 1 . IP/input ratios were calculated and normalized relative to ratios of IgG IPs. GUS histochemical staining GUS activity was detected using histochemical staining as previously described (Pichon et al. [66] ; roots were incubated for 3 h at 37 °C). After staining, roots were washed twice in sterile water and observed in bright field using an AxioZoom V16 macroscope (Zeiss, https://www.zeiss.fr ) or a Leica DM550 B (Leica Microsystems). Root sections were included in 3% agarose and then sliced into 80-µm sections using a VT 1200S vibratome (Leica Microsystems, http://www.leica-microsystems.com/ ). Vibratome sections mounted in water were observed in bright field using with an Olympus BX53 microscope ( www.olympus-lifescience.com ). Statistical analyses At least three independent biological replicates were performed in all experiments. Mann–Whitney non-parametric test, available in the Xlstat software ( http://www.xlstat.com/ ), was used to assess significant differences. To compare proportions of roots showing different GUS expression patterns, Fisher exact test was used. 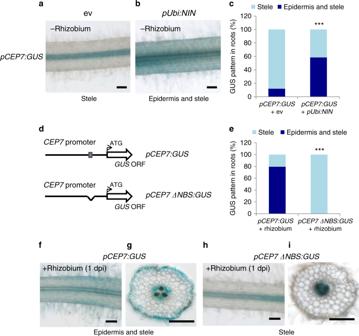Fig. 5: The NIN-binding sitecis-element predicted in the proximal region of theCEP7promoter is required for its induction by rhizobia. a–cNINexpression driven by thepUbipromoter is sufficient to induce the expression of aMtCEP7:GUSfusion in the absence of rhizobium (b), compared to an empty vector (ev) control (a). Representative images of theGUSexpression pattern associated only with the root stele (“stele”) or with both the root epidermis and stele (“epidermis and stele”). Wild-type plants were grown in vitro on a nitrogen-free Fåhraeus medium. In c, quantification of the proportion of roots (n≥ 25) showing aGUSexpression pattern associated only with the root stele or with both the root epidermis and stele, as described ina,b.d–hThe NIN-binding site (NBS) in the proximal region of theMtCEP7promoter is required for the induction of aMtCEP7:GUSfusion in response to rhizobium. Ind, schematic representation of theMtCEP7promoter, highlighting the predicted NBScis-element identified as a red box and the corresponding deletion construct (pCEP7ΔNBS:GUS). Ine, quantification of the proportion of roots (n≥ 34) showing aGUSexpression pattern associated only with the root stele (“stele”) or with both the root epidermis and stele (“epidermis and stele”), as described inf–i. Inf,g, representative images of theGUSexpression pattern associated only with the root stele or with both the root epidermis and stele ofpCEP7ΔNBS:GUS1 day post rhizobium inoculation (dpi) in longitudinal (f) or transversal (g) sections. Inh,i, representative images for the sameGUSexpression patterns forMtCEP7:GUSroots 1 dpi in longitudinal (h) or transversal (i) sections. Ina,b,f–i, a minimum of eight independent roots were analyzed for each time point from three independent experiments. Images show the GUS staining as a blue signal in bright field microscopy. Scale bars = 100 µm. Inc,e, Fisher exact test was performed to assess significant differences in the proportion of roots (n≥ 25) showing the differentGUSexpression patterns between the NIN overexpressing (c), or NBS-deletedMtCEP7:GUS(e) roots, and the control, as indicated by asterisks (***α< 0.001). 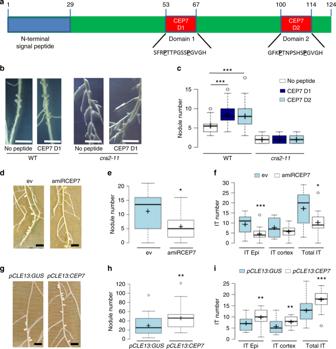Fig. 6: CEP7 peptides regulate positively nodule number and rhizobial infections. aSchematic representation of the predicted MtCEP7 prepropeptide. The blue rectangle represents the N-terminal signal peptide predicted using SignalP 3.0 (http://www.cbs.dtu.dk/services/SignalP-3.0/). Red rectangles represent the predicted MtCEP7 Domain 1 (CEP7 D1) and Domain 2 (CEP7 D2) peptide sequences with hydroxyl modifications to proline as indicated in bold.bRepresentative images of the nodulation phenotype of wild-type (WT) andcra2mutants treated with synthetic CEP7 D1 or CEP7 D2. Scale bars = 1 cm.cQuantification of the nodule number in WT andcra2mutants, grown in vitro on a nitrogen-free Fåhraeus medium supplemented or not with 1 µM CEP7 D1 or CEP7 D2 peptides. Nodule number was scored at 14 days post rhizobium inoculation (dpi). Graphs are based on data points from three biological replicates (n≥ 59). Mann–Whitney test was used for each genotype to assess significant differences between peptide-treated and control plants, as indicated by asterisks (***α< 0.001).dThe nodulation phenotype of plants expressing an artificial microRNA targetingMtCEP7transcripts (amiRCEP7). Representative images of nodulated roots transformed either with an empty vector (ev) or with the amiRCEP7 construct described ind. Scale bars = 1 cm.eQuantification of the nodule number of plants transformed either with an ev or with an amiRCEP7 construct. Plants were grown in vitro on a nitrogen-free Fåhraeus medium and nodules were scored at 14 dpi. Graphs are based on data points from 1 representative biological replicate out of 3 (n≥ 14). Mann–Whitney test was used to assess significant differences, as indicated by asterisks (*α< 0.05).fQuantification of infection thread (IT) number in six dpi roots transformed either with an ev or with the amiRCEP7 construct and inoculated with a rhizobium strain constitutively expressing a LacZ reporter. ITs that reached the epidermis (epidermal ITs) were distinguished from ITs that reached the cortex (cortical ITs). Graphs are based on data points from two biological replicates (n≥ 15). Mann–Whitney test was used to assess significant differences between amiRCEP7 roots and control roots, as indicated by asterisks (*α< 0.05; ***α< 0.001).gRepresentative images of the nodulation phenotype of plants transformed either with apCLE13:GUSor apCLE13:CEP7construct. Scale bars = 1 cm.hQuantification of the nodule number in plants transformed either with thepCLE13:CEP7construct or thepCLE13:GUSconstruct as a negative control. Plants were grown in pots containing a perlite/sand (3/1) mixture and watered with a “i” low nitrogen medium, and nodules were scored at 21 dpi. Graphs are based on data points from two biological replicates (n≥ 28). Mann–Whitney test was used to assess significant differences, as indicated by asterisks (**α< 0.01).iQuantification of IT number in six dpi roots transformed either with thepCLE13:CEP7construct or thepCLE13:GUSconstruct as a negative control and inoculated with a rhizobium strain constitutively expressing a LacZ reporter. ITs that reached the epidermis (epidermal ITs) were distinguished from ITs that reached the cortex (cortical ITs). Graphs are based on data points from two biological replicates (n≥ 15). Mann–Whitney test was used to assess significant differences between thepCLE13:CEP7roots and control roots, as indicated by asterisks (**α< 0.01; ***α< 0.001). Inc,e,f,h,i, center lines show the medians; box limits indicate the 25th and 75th percentiles as determined by the R software; whiskers extend 1.5 times the interquartile range from the 25th and 75th percentiles, outliers are represented by dots; and crosses represent sample means. Accession numbers Sequence data from this article were retrieved from the M. truncatula genome v4.0 ( https://phytozome.jgi.doe.gov/ ; Tang et al. [67] ) and/or the M. truncatula genome v5 ( https://medicago.toulouse.inra.fr/MtrunA17r5.0-ANR/ ; Pecrix et al. [68] ) under the following accession numbers, respectively: MtCLE13 , Medtr4g079610.1 or MtrunA17Chr4g0040951; MtCRA2 , Medtr3g110840.1 or MtrunA17Chr3g0140861; MtCRE1 , Medtr8g106150.1 or MtrunA17Chr8g0392301, MtNIN , Medtr5g099060 or MtrunA17Chr5g0448621; MtCEP7 , MtrunA17Chr8g0374811. The MtCEP7 sequence, absent from the v4.0 version, was alternatively retrieved from the M. truncatula v3.5 database (AC233112_1013; http://blast.jcvi.org/Medicago-Blast ). Reporting summary Further information on research design is available in the Nature Research Reporting Summary linked to this article.